Epidermal photonic devices for quantitative imaging of temperature and thermal transport characteristics of the skin Characterization of temperature and thermal transport properties of the skin can yield important information of relevance to both clinical medicine and basic research in skin physiology. Here we introduce an ultrathin, compliant skin-like, or ‘epidermal’, photonic device that combines colorimetric temperature indicators with wireless stretchable electronics for thermal measurements when softly laminated on the skin surface. The sensors exploit thermochromic liquid crystals patterned into large-scale, pixelated arrays on thin elastomeric substrates; the electronics provide means for controlled, local heating by radio frequency signals. Algorithms for extracting patterns of colour recorded from these devices with a digital camera and computational tools for relating the results to underlying thermal processes near the skin surface lend quantitative value to the resulting data. Application examples include non-invasive spatial mapping of skin temperature with milli-Kelvin precision (±50 mK) and sub-millimetre spatial resolution. Demonstrations in reactive hyperaemia assessments of blood flow and hydration analysis establish relevance to cardiovascular health and skin care, respectively. Spatio-temporal imaging of skin temperature offers experimental and investigational value in many areas of medicine, such as for detection of breast cancers and other syndromes, as an adjunctive screening tool to mammography [1] , [2] , [3] . The required milli-Kelvin levels of precision and millimetre-scale resolution are most commonly achieved by the use of sophisticated infrared digital imaging cameras. However, widespread adoption of such technology is limited by high capital costs, motion artefacts and inability for use outside of clinical or laboratory settings. Other low-cost thermography techniques have been explored for potential screening of deep venous thrombosis [4] , [5] , [6] , [7] , breast cancer [8] , [9] , [10] , spinal root syndromes [11] , [12] , chronic back pain [13] and even pulmonological diagnostics [14] . Recent work [15] , [16] demonstrates that electronic temperature-mapping devices can be constructed in ultra-thin, soft and compliant formats, sometimes referred to as ‘epidermal’ due to the similarity of their physical characteristics to those of the skin itself. These systems offer capabilities that bypass many limitations of infrared cameras, but provide only modest spatial resolution and imaging fidelity, limited by multiplexing systems needed to address large sensor arrays. Untethered, wireless operation also demands data transmission components and power sources. Other stretchable smart skin devices that can monitor the vital health signals of the wearer with high levels of function and comfort have been investigated intensively [15] , [17] , [18] , [19] , [20] , [21] , [22] , [23] , [24] , [25] . Here we introduce a simple alternative that combines colorimetric readout and radio frequency (RF) actuation for mapping of thermal characteristics of the skin. The sensors exploit thermochromic liquid crystals (TLC) patterned into large-scale, pixelated arrays on thin elastomeric substrates. Co-integration with electronics provides a means for controlled, local heating by RF signals, to enable not only mapping of temperature but also intrinsic thermal constitutive properties. Uniform layers of TLCs in water-impermeable, non-stretchable thick plastic sheaths, and without electronics, have been explored for skin thermography [26] , [27] , [28] but without the ability to conform sufficiently well to the curved, textured surface of the skin for accurate, reproducible measurements. Such devices also frustrate transepidermal water loss. They also thermally load the skin and cause irritation at the skin interface, thereby preventing reliable, accurate evaluation or use in continuous modes over long periods of time. Thermochromic textiles are available for cosmetic and fashion purposes [29] , [30] , [31] but their inability to maintain intimate contact with the skin and the limited capacity to use known thermochromic dyes for precision temperature evaluation prevent their use in the sorts of applications envisioned here. The devices reported in this paper not only avoid these drawbacks but they also allow precise measurement of thermal conductivity and thermal diffusivity through analysis of spatio-temporal images obtained during operation of integrated RF components. Conventional digital cameras and RF transmission systems enable simultaneous readout of thousands of pixels at resolutions that exceed those needed to image temperature and thermal property variations on the skin. The epidermal format induces minimal perturbations on the natural mechanical and thermal properties of the skin. Results presented in the following establish the foundational aspects in materials, mechanics and thermal physics for both electronically active and passive epidermal TLC (e-TLC) devices, including algorithms for extracting precision, calibrated data from colour digital images. Demonstrations in reactive hyperaemia assessments of blood flow, as it relates to cardiovascular health, and hydration analysis, as it relates to skin-care, provide two examples of use in clinically meaningful tests. Design and fabrication The e-TLC thermal imagers use a multilayer design that includes a thin (20 μm) black elastomeric membrane as a mechanical support and an opaque background for accurate colorimetric evaluation of the TLC materials; an array of dots of TLC (that is, pixels with 25 μm thicknesses and diameters of either 250 or 500 μm, spaced by 250 or 500 μm), with an optional interspersed array of dots with fixed colours (with 25 μm thicknesses, diameters of 400 μm, spaced by 600 μm) for calibration, both delivered to the surface of the black elastomer by transfer printing; a thin (30 μm) overcoat of a transparent elastomer for encapsulation and optional electronics in thin, stretchable configurations mounted on the back surface for active functionality described subsequently (details appear in Supplementary Fig. 1 and Supplementary Note 1 ). The TLC material consists of microencapsulated chiral nematic liquid crystals. With increasing temperature, the phase varies from crystalline solid to smectic, cholesteric and, finally, isotropic liquid, all over a range of a few degrees, dictated by the chemistry [32] , [33] . In the cholesteric phase, light that reflects from the TLC pixels spans a narrow wavelength range defined by phase coherent interactions with the liquid crystal assemblies. Increases in temperature decrease the pitch, thereby leading to blueshifts in the peak wavelengths of this reflected light. This behaviour provides the basis for colorimetric optical readout. Other phases have no chiral nematic orientation of molecular planes and, thus, do not yield any strong wavelength dependence to the reflection. The small sizes and large spacings of the TLC and calibration pixels, taken together with the low modulus, elastic properties of the substrate, encapsulation layer and electronics, yield soft, compliant mechanics in the overall e-TLC system. These properties yield devices that are well suited for mounting on the skin. 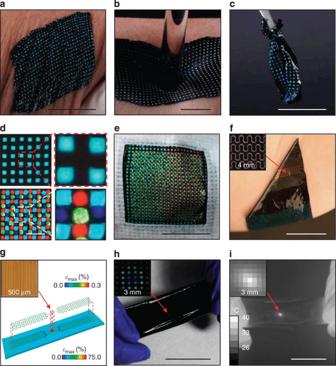Figure 1: e-TLC thermal imaging device as an example of an epidermal photonic system. (a) Picture of a device on the skin deformed by pinching in a twisting motion. Scale bar, 3 cm. (b) Picture of a device deformed by poking with a warm glass rod while on the skin. Scale bar, 1 cm. (c) Picture of a device collapsed under its own weight while free-standing. Scale bar, 2 cm. (d) Magnified view of a device operating in the blue region of the spectrum, without and with integrated patterns of dots that have fixed colours for calibration. Scale bar, 2 mm. (e) Picture of a device with calibration colours operating on the curved surface of the skin. Scale bar, 2 cm. (f) Picture of a device that includes a RF antenna and Joule heating element on its back surface, folded over and resting on the palm, with an enlarged view of the serpentine antenna structure (inset). Scale bar, 2 cm. (g) Schematic illustration of finite element modelling results for a device with wireless heater under tensile strain, with magnified view of the Joule heating element (inset). (h) Image of an active, wireless device collected while exposed to RF power in air, with magnified view of the colour changes induced by the heater (inset). Scale bar, 3 cm. (i) Infrared image of the same device under similar conditions, with magnified view in the region of the heater (inset). Scale bar, 3 cm. Figure 1a–c shows an e-TLC device on the skin of the forearm when twisted and gently poked with a mildly heated rod. Low interfacial stresses that follow from the low effective modulus and small thickness of the device enable adequate adhesion through van der Waals interactions alone. The collapse of a free-standing device under its own weight, as in Fig. 1c , provides qualitative evidence of these mechanical characteristics. Figure 1d shows a pair of magnified images of e-TLC devices; those on the bottom include interspersed colour calibration pixels consisting of red, green and blue dye in a non-toxic acrylic base (aqueous dispersion of organic pigment and acrylic polymer, Createx). A completed device of this latter type placed on the curved surface of the back of the hand appears in Fig. 1e . As previously mentioned, the backside of the black elastomer substrate provides a mounting location for stretchable electronics. The image in Fig. 1f shows an example of an e-TLC device with a wireless system integrated in this way, for remote delivery of controlled levels of heat. The folded configuration reveals part of the serpentine antenna structure (inset). An illustration of this system, in the form of three-dimensional finite element analysis (3D-FEA), appears in Fig. 1g . The antenna captures incident RF energy to power a Joule heating element (inset, Fig. 1g ). The result provides well-defined, localized increases in temperature, as revealed in the pattern of colours in the TLC pixels of Fig. 1h and the infrared images of Fig. 1i . As described subsequently, the results from measurements under such conditions allow determination of the thermal conductivity and thermal diffusivity of the skin. Figure 1: e-TLC thermal imaging device as an example of an epidermal photonic system. ( a ) Picture of a device on the skin deformed by pinching in a twisting motion. Scale bar, 3 cm. ( b ) Picture of a device deformed by poking with a warm glass rod while on the skin. Scale bar, 1 cm. ( c ) Picture of a device collapsed under its own weight while free-standing. Scale bar, 2 cm. ( d ) Magnified view of a device operating in the blue region of the spectrum, without and with integrated patterns of dots that have fixed colours for calibration. Scale bar, 2 mm. ( e ) Picture of a device with calibration colours operating on the curved surface of the skin. Scale bar, 2 cm. ( f ) Picture of a device that includes a RF antenna and Joule heating element on its back surface, folded over and resting on the palm, with an enlarged view of the serpentine antenna structure (inset). Scale bar, 2 cm. ( g ) Schematic illustration of finite element modelling results for a device with wireless heater under tensile strain, with magnified view of the Joule heating element (inset). ( h ) Image of an active, wireless device collected while exposed to RF power in air, with magnified view of the colour changes induced by the heater (inset). Scale bar, 3 cm. ( i ) Infrared image of the same device under similar conditions, with magnified view in the region of the heater (inset). Scale bar, 3 cm. Full size image Mechanical and thermal analysis A key design goal is to produce e-TLC systems that induce minimal perturbations to the skin, thereby avoiding irritation, enhancing wearability and ensuring accurate measurement capabilities. The mechanical and thermal properties are particularly important in this context. Experimental and theoretical studies of the former reveal low modulus, elastic characteristics over large ranges of strain. 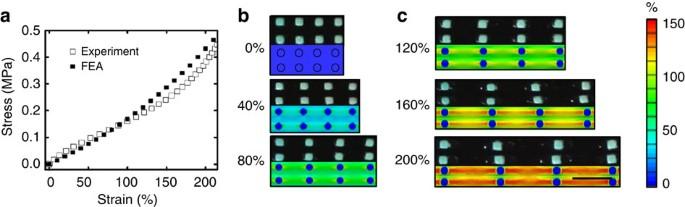Figure 2: Mechanical properties of e-TLC devices. (a) Measurements and theoretical calculations of stress–strain responses of a device. (b) Comparison between images and three-dimensional finite element modelling of a representative region of e-TLC device under different levels of tensile strain. Scale bar, 2 mm. Figure 2a shows the stress/strain responses of an e-TLC device under static uniaxial testing. The results agree well with the predictions of 3D-FEA. In particular, the TLC pixels (~221 MPa) and elastomeric substrate (~131 kPa) yield an effective modulus (~152 kPa and 178 kPa from 3D-FEA and experiment, respectively) that is only slightly larger (by 16–35%) than the intrinsic value associated with the bare elastomer, and is comparable to that of the epidermis itself. The TLC pixels experience ultra-low strain (for example, <2%) even under extreme stretching (for example, 200%), as shown in Fig. 2b . Negligible deformations of the TLC pixels, as observed in experiment and FEA ( Fig. 2b ), allow approximations for simple, but quantitatively accurate, analytical solutions of the mechanics (see Supplementary Note 2 and Supplementary Fig. 2a ). The thicknesses, bending stiffnesses, effective moduli and stretchability of these devices are 50 μm, 3.0 nN m, 178 kPa and beyond 200%, respectively; these characteristics are superior than those of typical, commercially available TLC sheets (Feverscan, Hallcrest) whose corresponding properties are of ~125 μm, 570,000 nN m, 3.3 GPa and ~5%, respectively. The differences are significant at a qualitative level of importance for deployment on the skin. In particular, the collective mechanical characteristics allow largely unconstrained natural motions of the skin, including wrinkling and stretching, even in challenging regions such as the knees and elbows. Addition of calibration pixels reduces the stretchability and increases the modulus ( Supplementary Fig. 2b ), but retain elastic behaviours at strain levels (50%) that exceed those that can be tolerated by the epidermis (linear response to tensile strain up to 15%, nonlinear to 30% and rupture at >30% (ref. 34 )). Incorporating a wireless electronic heating system further reduces the accessible strain, but with an elastic stretchability of nearly 20%, which is useful for many applications (see Supplementary Fig. 3 ) [35] , [36] . Although the characteristics of the antenna change with mechanical deformation, experiments indicate that uniaxial stretching (up to 50%) does not disrupt the overall function or the efficiency of power harvesting (see Supplementary Fig. 4 ); bending can decrease the efficiency. The thermal characteristics of the systems define the thermal load on the skin, as well as the overall time response. For an active e-TLC device, the thermal mass per unit area is ~7.7 mJ cm −2 K −1 ( Supplementary Note 3 ). This value corresponds to an equivalent of skin with thickness of ~20 μm, that is, only 25% of the thickness of the epidermis itself [37] . Water vapour permeability tests on e-TLC and Feverscan strip devices ( Supplementary Note 4 and Supplementary Fig. 5 ) reveals that e-TLC devices provide only minor moisture barrier for operation on the skin. Decreasing the thickness of the device increases the water permeation, as expected (see Supplementary Fig. 5b ). Additional increases can be achieved by microstructuring, that is, introducing arrays of holes or pores. The small thermal mass and high water permeability minimize changes in skin temperature and hydration level induced by the presence of the device. Temperatures measured with an infrared camera on the forearm adjacent to an e-TLC and directly underneath it ( Supplementary Fig. 6a–c ) show minimal differences. The effects of the device on skin hydration ( Supplementary Fig. 6d,e ) are also small. A mounted 80-μm-thick e-TLC on well-hydrated skin (~35) leads to a small percentage increase in hydration (7.5%) after 3 h. For an otherwise identical set of testing conditions, the Feverscan strip led to a ~100% increase in hydration. For monitoring of transient processes, the time response of the system is important. With geometries and materials investigated here, the response time for an e-TLC device is dominated by the thickness and thermal properties of the black elastomer substrate. Transient measurements reveal response times of less than ~30 ms ( Supplementary Note 5 ), consistent with estimates developed using analytical models ( Supplementary Fig. 7 ). The intrinsic switching times for most TLC materials are ~3–10 ms (refs 38 , 39 , 40 , 41 ). Figure 2: Mechanical properties of e-TLC devices. ( a ) Measurements and theoretical calculations of stress–strain responses of a device. ( b ) Comparison between images and three-dimensional finite element modelling of a representative region of e-TLC device under different levels of tensile strain. Scale bar, 2 mm. Full size image Optical and image analysis Reflection mode spectroscopic characterization (Zeiss Axio Observer D1) of the steady-state response of the TLC material to changes in temperature between 32 °C and 39 °C show expected behaviours, as in Fig. 3a . With proper calibration, described next, the temperature extracted from the hue and saturation values determined using a typical digital camera (Canon 5D Mark II) with the e-TLC device held at a nominally constant temperature exhibits an s.d. of ~30 mK over a measurement time of 760 s. This value is comparable to that observed from temperature readings simultaneously determined with an infrared camera (~50 mK) ( Fig. 3b ). The measurement precision is, then, at least ±50 mK under these experimental conditions. Equivalent temperatures extracted from analysis of colour recorded at the calibration pixels (red, green and blue) show fluctuations with similar magnitudes, as summarized in Fig. 3c . These observations suggest that the process of image capture and colour analysis enables levels of precision that are comparable to those of infrared cameras, not limited by the physics of the TLC. Detailed calibration plots and information on temperature extraction appear in Supplementary Fig. 8 . 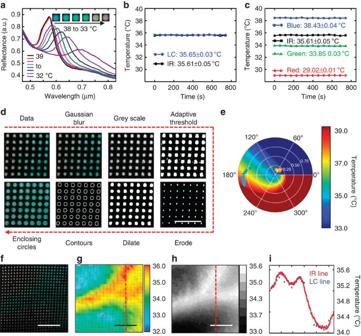Figure 3: Calibration and use of e-TLC devices for skin thermal imaging. (a) Reflectance measured at a single pixel from 32 °C to 39 °C and corresponding images for 33 °C to 38 °C (inset). (b) Temporal variations in temperature extracted from digital colour analysis of an e-TLC held, nominally, at a constant temperature. (c) Temporal variations in apparent temperature determined from colour analysis of calibration pixels in an e-TLC device. Framesbandcalso show results obtained with an infrared camera. (d) Illustration of the steps for processing digital images of e-TLC devices, demonstrated on a representative 7 × 7 array of pixels. Scale bar, 5 mm. (e) Colour–temperature calibration determined using hue analysis. (f) Images of an e-TLC device that consists of an 26 × 26 array of pixels, conformally mounted on the wrist. Scale bar, 1 cm. (g) Three-dimensional rendering of the temperature distribution extracted from the colour information obtained by hue value analysis of digital images of the device. Scale bar, 1 cm. (h) Two-dimensional rendering of temperature captured by an infrared camera at the same time and at the same location as ing. Scale bar, 1 cm. (i) Line-cut temperature profiles extracted from the data ofgandh. Figure 3: Calibration and use of e-TLC devices for skin thermal imaging. ( a ) Reflectance measured at a single pixel from 32 °C to 39 °C and corresponding images for 33 °C to 38 °C (inset). ( b ) Temporal variations in temperature extracted from digital colour analysis of an e-TLC held, nominally, at a constant temperature. ( c ) Temporal variations in apparent temperature determined from colour analysis of calibration pixels in an e-TLC device. Frames b and c also show results obtained with an infrared camera. ( d ) Illustration of the steps for processing digital images of e-TLC devices, demonstrated on a representative 7 × 7 array of pixels. Scale bar, 5 mm. ( e ) Colour–temperature calibration determined using hue analysis. ( f ) Images of an e-TLC device that consists of an 26 × 26 array of pixels, conformally mounted on the wrist. Scale bar, 1 cm. ( g ) Three-dimensional rendering of the temperature distribution extracted from the colour information obtained by hue value analysis of digital images of the device. Scale bar, 1 cm. ( h ) Two-dimensional rendering of temperature captured by an infrared camera at the same time and at the same location as in g . Scale bar, 1 cm. ( i ) Line-cut temperature profiles extracted from the data of g and h . Full size image Analysis of hue/saturation/value (HSV) data obtained from the digital camera represents the simplest and most straightforward analysis approach. Sophisticated algorithms based on computer vision techniques are advantageous, however, not only for colour determination but for full pixelated analysis of complete e-TLC devices. Figure 3d illustrates an example of a process that exploits computer vision code (OpenCV), in which an image of an e-TLC device that consists of a 7 × 7 pixel array undergoes a set of colour extraction and data transformation steps (details in Supplementary Note 6 ). A Gaussian filter first reduces noise through smoothing to yield a grey scale rendering for use with an adaptive threshold that compensates for illumination non-uniformities. The output is a binary mask containing value ‘1’ at bright areas and ‘0’ elsewhere. A two-step erode/dilate process eliminates small speckles that arise from defects. A full list of contours can be extracted from this ‘clean’ image, in which each contour bounds a single pixel in the array. An enclosing circle function uses the contours as inputs to define the pixel positions, for extraction of colour information from the original, unprocessed image. A typical calibration that relates hue and saturation values extracted in this manner to temperature evaluated with an infrared camera appears in Fig. 3e . The biggest advantage of using HSV colour space instead of red/green/blue is that the colour information is encoded only in two (hue and saturation), rather than three (red, green and blue) channels. These two values are comparatively resilient to changes in lightning levels since that information is stored separately in the value channel. Any possible hue/saturation combination can be represented by a point in polar coordinates where radial coordinate corresponds to saturation and angular one to hue. The positions of the calibration set are marked with the dots painted with the corresponding hue. These points define the temperature calibration surface by means of two-dimensional linear fit. The results allow any hue/saturation combination to be assigned to a temperature value, as indicated in the plot using a colour gradient. Scaled use of this process is summarized in Fig. 3f . Here, a full e-TLC device on a portion of the wrist where near-surface veins are located reveals corresponding variations in temperature of the epidermis. The hue values across the e-TLC yield three-dimensional temperature contour plots that reflect the blood vessels with high spatial resolution ( Fig. 3g ). A direct comparison with temperature distributions measured in the same region with an infrared camera ( Fig. 3h ) exhibits excellent agreement. Plots of the temperature extracted from these two sets of results at the locations indicated by the dashed red lines in Fig. 3g,h appear in Fig. 3i . These results suggest suitability of e-TLC systems for mapping of vascular distributions in applications such as screening for deep venous thrombosis, without the need for costly infrared camera systems. In such practical situations, the lighting conditions can strongly affect the precision and accuracy of the temperature determination [42] , [43] , [44] , [45] . In particular, the hue and saturation depend on the type of light source used for illumination. The colour calibration pixels provide a means to compensate for such effects, as their known colours are influenced by the lighting in the same way as the TLC. As a result, it should be possible to develop algorithms that account for shifts in the apparent colours of these calibration pixels and yield a set of numerical compensations that can restore their actual, known colours. Applying the same compensations to the TLC pixels will serve as the basis for a temperature evaluation process that is independent of illumination conditions, within some reasonable range. Effects of three different lightning conditions appear in Fig. 4 . Red, green and blue colour calibration pixels, interspersed across the entire device, are present in this active e-TLC sample. 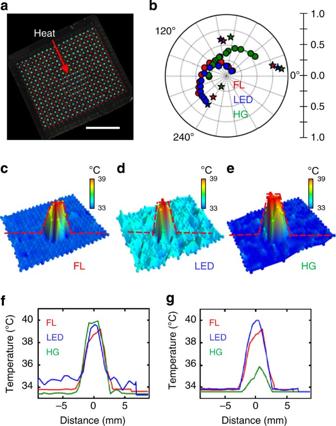Figure 4: Temperature analysis under different illumination conditions. (a) Image of a device immediately after local heating at the centre of the array. Scale bar, 1 cm. (b) Hue and saturation values extracted for the calibration (stars) and sensing pixels (dots; red—illumination with a fluorescent light (FL); blue—illumination with a light-emitting diode (LED); green—illumination with a halogen lamp (HG)). Three-dimensional rendering of colour-corrected temperatures determined with (c) white FL, (d) white LED, (e) HG. (f) Line graphs of results collected along the dashed lines shown inc–e. (g) Results similar to those inf, but with fluorescent temperature fit applied to all explored lightning conditions. Figure 4a presents an image of the device, with circles that indicate the positions of the TLC pixels. A Joule heating element is present in the centre region. Fluorescent, light-emitting diode and halogen ( Fig. 4c–e ) light sources provide a range of practical examples. The corresponding temperature calibration data appear in Fig. 4b . The circles correspond to the HSVs of TLC pixels recorded at different temperatures to define calibration fits for specific light sources. The stars delineate the effect of illumination on the colours of the calibration pixels. Red, green and blue calibration pixels are located at ~5°, ~100° and ~240°, respectively. As these colours are known, data from them allow extraction of compensation factors for any given lighting condition. Applying the results to measurements of TLC pixels dramatically reduces the sensitivity of the temperature detection process to the lightning source. Figure 4f presents computed temperatures evaluated along lines that pass through the central region while the Joule element is activated. The results are comparable for all three lighting sources. To demonstrate the importance of proper calibration, Fig. 4g summarizes data that exploit the fluorescent temperature fit for all lighting conditions explored here. Significant discrepancies occur, as might be expected due to the different colour temperatures of the halogen and light-emitting diode sources; these are reflected not only in the temperature maxima, but also the temperature profiles, shapes and noise levels, all of which again emphasizes the importance of proper calibration and potential for compensation approaches. Figure 4: Temperature analysis under different illumination conditions. ( a ) Image of a device immediately after local heating at the centre of the array. Scale bar, 1 cm. ( b ) Hue and saturation values extracted for the calibration (stars) and sensing pixels (dots; red—illumination with a fluorescent light (FL); blue—illumination with a light-emitting diode (LED); green—illumination with a halogen lamp (HG)). Three-dimensional rendering of colour-corrected temperatures determined with ( c ) white FL, ( d ) white LED, ( e ) HG. ( f ) Line graphs of results collected along the dashed lines shown in c – e . ( g ) Results similar to those in f , but with fluorescent temperature fit applied to all explored lightning conditions. Full size image Skin thermal property measurements As suggested by the active e-TLC results in Fig. 4 , the local Joule heating element enables additional measurement capabilities. In particular, spatial and temporal variations in temperature at locations near this heater can be used, with thermal models, to extract the thermal conductivity and diffusivity of the skin. Increases in temperature of a few °C can be sufficient for accurate evaluation. The thermal conductivity ( k ) can be determined by comparing measured steady-state distributions in temperature to axisymmetric thermal conduction models (see Supplementary Note 7 ). Calculations based on this model suggest spatial decays in temperature ( T sensor–layer ) that vary as 1/ r (except the central sensor), which can be written as where r is the distance from the heat source, Q is the heat generated by the Joule heating element and T ∞ is the temperature of surrounding air. An example appears in Fig. 5a , with details in Supplementary Fig. 9a,b,e . Calibration can be performed through measurements of materials with known properties ( Fig. 5b ). 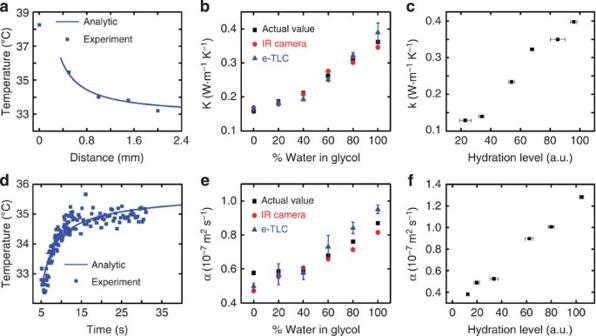Figure 5: Determination of skin thermal conductivity and thermal diffusivity. (a) Example of temperatures (symbols) as a function of distance from the position of local heating in an active e-TLC device and corresponding best-fit modelling results (analytic; line) for determining the thermal conductivity. (b) Thermal conductivity of water/ethylene glycol solutions evaluated using an active e-TLC device, and comparison with values obtained from the literature and from analysis of temperatures determined with an infrared camera. The error bars represent average s.d. of measurements obtained with e-TLC, which is ≤9%. (c) Thermal conductivities measured with an active e-TLC device on the skin at different levels of hydration, separately measured with a commercial moisture meter. The error bars represent average s.d. of measurements obtained with the moisture meter. (d) Example of temperatures (symbols) as a function of time for a location near a wireless heater in an active e-TLC device, and corresponding best-fit modelling results (analytic; line) for determining the thermal diffusivity. (e) Thermal diffusivity of water/ethylene glycol solutions evaluated using an active e-TLC device, and comparison with values obtained from the literature and from analysis of temperatures determined with an infrared camera. The error bars represent average s.d. of measurements obtained with e-TLC, which is ≤14%. (f) Thermal diffusivities measured with an active, wireless e-TLC device on the skin at different levels of hydration, separately measured with a commercial moisture meter. The error bars represent average s.d. of measurements obtained with the moisture meter. Figure 5c indicates excellent correspondence between thermal conductivity of the skin evaluated with an active e-TLC and hydration levels determined with a moisture meter (Delfin MoistureMeterSC) that relies on electrical impedance. The quantitative values of k fall within a range that is consistent with literature values determined by subcutaneous thermocouples and high-speed radiometers [46] . By simplifying the heating element as a point heat source that turns on at time t =0, the transient temperature variation can be analytically solved as (see Supplementary Note 8 ) Figure 5: Determination of skin thermal conductivity and thermal diffusivity. ( a ) Example of temperatures (symbols) as a function of distance from the position of local heating in an active e-TLC device and corresponding best-fit modelling results (analytic; line) for determining the thermal conductivity. ( b ) Thermal conductivity of water/ethylene glycol solutions evaluated using an active e-TLC device, and comparison with values obtained from the literature and from analysis of temperatures determined with an infrared camera. The error bars represent average s.d. of measurements obtained with e-TLC, which is ≤9%. ( c ) Thermal conductivities measured with an active e-TLC device on the skin at different levels of hydration, separately measured with a commercial moisture meter. The error bars represent average s.d. of measurements obtained with the moisture meter. ( d ) Example of temperatures (symbols) as a function of time for a location near a wireless heater in an active e-TLC device, and corresponding best-fit modelling results (analytic; line) for determining the thermal diffusivity. ( e ) Thermal diffusivity of water/ethylene glycol solutions evaluated using an active e-TLC device, and comparison with values obtained from the literature and from analysis of temperatures determined with an infrared camera. The error bars represent average s.d. of measurements obtained with e-TLC, which is ≤14%. ( f ) Thermal diffusivities measured with an active, wireless e-TLC device on the skin at different levels of hydration, separately measured with a commercial moisture meter. The error bars represent average s.d. of measurements obtained with the moisture meter. Full size image where α is the thermal diffusivity of the skin and erfc ( x ) is the complementary error function. Therefore, transient temperature data associated with activation or deactivation of the Joule heating element can be used to determine thermal diffusivity, α , as illustrated in Fig. 5d (see Supplementary Fig. 9a,b,f ). As with conductivity, the device can be calibrated using samples with known diffusivity ( Fig. 5e ). Here, a wireless active e-TLC system serves as the measurement vehicle. The time dependence of the temperature, rather than the absolute values, is sufficient for extraction of diffusivity. The device operates at frequencies of ~2 GHz with maximum power inputs of ~2.5 W kg −1 for the subject of the studies described here (that is, one-third of the power limit recommended by the Federal Communications Commission’s guidelines). The results correspond closely to the hydration level, as shown in Fig. 5f . As with k , the values of α are consistent with literature reports based on techniques such as opto-thermal measurement [47] . The values of k and α can be combined to yield the product of the density ( ρ ) and heat capacity ( c ) of the skin, based on the relation ( cρ = k / α ). The calculations (see Supplementary Fig. 9g ) show that the heat capacity increases slightly with hydration level (assuming that ρ is approximately constant), which is consistent with expectation, as the heat capacity (~4.2 J g −1 K −1 ) of water is larger than the human tissue (for example, ~3.7 J g −1 K −1 for the dermis and ~2.3 J g −1 K −1 for fat) [48] . Spatio-temporal mapping of reactive hyperaemia test Spatio-temporal mapping even with passive e-TLC systems yields useful information on blood circulation [49] , [50] , maximal percentage increase in blood flow rate after occlusion [51] and duration of reactive hyperaemia [52] . Measurements of temperature fluctuations above the ulnar artery and adjacent veins serve as an important part of a reactive hyperaemia protocol. Here, the flow of blood is temporarily occluded by a pressure cuff on the upper arm, followed by abrupt release. 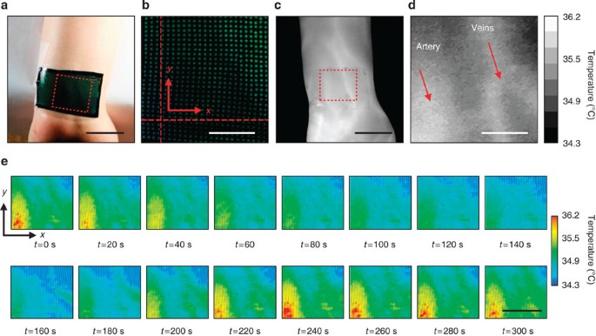Figure 6: Application of an e-TLC device in a reactive hyperaemia test. (a) Optical images of an e-TLC device on the wrist during an occlusion test. Scale bar, 3 cm. (b) Magnified view of the device in a. Scale bar, 1 cm. (c) Infrared image of e-TLC device on the wrist. Scale bar, 3 cm. (d) Magnified view of the device inc. Scale bar, 1 cm. (e) Three-dimensional rendering of spatial distributions of temperature determined with the e-TLC device at different times during and after occlusion (occlusion starts att=0 s and ends att=160 s). Scale bar, 2 cm. Figure 6a–d summarizes results of measurements performed with an e-TLC device and an infrared camera. Figure 6e presents representative frames of temperature distributions captured at 20 s intervals throughout the experiment. Occlusion, which begins at t =0 s, causes the temperature of the skin above the ulnar artery and adjacent areas to decrease drastically, owing to lack of incoming blood flow and loss of heat to the environment. The minimum temperature is achieved at t =160 s; at this time, the occlusion is released and blood flow resumes. Sharp temperature increases occur in areas above the blood vessels, as shown in Fig. 6e , until the temperature stabilizes. The responses of pixels across the array of the e-TLC vary widely depending on their distance from the blood vessels. The maximum temperature fluctuations are ~1.2 °C and occur immediately above the ulnar artery; the minimum temperature fluctuations are ~0.4 °C and occur at locations away from near-surface blood vessels. Direct comparisons of spatio-temporal variations in temperature obtained from the e-TLC show quantitative agreement with results from an infrared camera ( Supplementary Fig. 10 ). 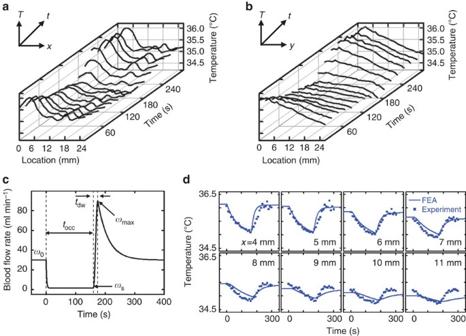Figure 7: Study of thermal processes in a reactive hyperaemia test. (a) Line graphs of temperatures along the horizontal dashed red line in Fig. 6b, at various times. (b) Line graphs of temperatures along the vertical dashed red line in Fig. 6b, at various times. (c) Rate of blood flow through the ulnar artery determined by comparison of thermal models with experimental results. The key parameters include: the occlusion time (tocc)=160 s; time-to-peak-flow (tdw)=15 s; the baseline flow rate (ω0)=30 ml min−1; the occluded flow rate (ωs)=1.5 ml min−1; and the peak flow rate (ωmax)=90 ml min−1. (d) Measured temperature rise at the surface of the skin above the ulnar artery during the occlusion along with results from finite element analyses (FEA) using the blood flow rate in framec. The eight sub-frames correspond to the temperature histories of different points at the horizontal dashed red line inFig. 6b. Figure 7a,b highlights temperature variations along horizontal and vertical lines illustrated in Fig. 6b . A thermal model of the human wrist ( Supplementary Note 9 , Supplementary Tables 1 and 2 , and Supplementary Fig. 11 ) that accounts for both the time–dynamic effect of occlusion and the thermal diffusion from the ulnar artery can capture the effects revealed in the measurements ( Fig. 7c,d ) and enable extraction of additional physiological information. The temporal variation of blood flow can be described with a piecewise, exponential type function [53] , [54] , corresponding to the three stages of the process: pre-occlusion, vascular occlusion and reperfusion. The parameters characterizing this piecewise function can be determined by minimizing the average differences between the temperature–time profiles predicted by the model and those measured by the e-TLC device, during each stage. Figure 7d shows that the calculated temperature history based on the thermal model agrees with experiment at all six of the pixels near the artery (that is, distance <6 mm). Owing to simplifying assumptions in the models, the FEA does not quantitatively capture the overshoot behaviour observed in the two nearest sensors. Discrepancies at the two most distant sensors can be attributed to the neglect of heating associated with a nearby vein (~13 mm from the artery) in the model. For vessel diameters and depths that lie within reported ranges ( Supplementary Note 9 ), the peak blood flow velocity after occlusion is calculated to be 58.8 cm s −1 , representing a threefold increase over the baseline of 19.6 cm s −1 , with reactive hyperaemia duration of 144 s. These values match those reported in the literature for a person with low cardiovascular risk [51] , [52] . Figure 6: Application of an e-TLC device in a reactive hyperaemia test. ( a ) Optical images of an e-TLC device on the wrist during an occlusion test. Scale bar, 3 cm. ( b ) Magnified view of the device in a. Scale bar, 1 cm. ( c ) Infrared image of e-TLC device on the wrist. Scale bar, 3 cm. ( d ) Magnified view of the device in c . Scale bar, 1 cm. ( e ) Three-dimensional rendering of spatial distributions of temperature determined with the e-TLC device at different times during and after occlusion (occlusion starts at t =0 s and ends at t =160 s). Scale bar, 2 cm. Full size image Figure 7: Study of thermal processes in a reactive hyperaemia test. ( a ) Line graphs of temperatures along the horizontal dashed red line in Fig. 6b, at various times. ( b ) Line graphs of temperatures along the vertical dashed red line in Fig. 6b, at various times. ( c ) Rate of blood flow through the ulnar artery determined by comparison of thermal models with experimental results. The key parameters include: the occlusion time ( t occ )=160 s; time-to-peak-flow ( t dw )=15 s; the baseline flow rate ( ω 0 )=30 ml min −1 ; the occluded flow rate ( ω s )=1.5 ml min −1 ; and the peak flow rate ( ω max )=90 ml min −1 . ( d ) Measured temperature rise at the surface of the skin above the ulnar artery during the occlusion along with results from finite element analyses (FEA) using the blood flow rate in frame c . The eight sub-frames correspond to the temperature histories of different points at the horizontal dashed red line in Fig. 6b . Full size image Epidermal photonic systems, as embodied by the e-TLC devices introduced here, offer strong potential for characterization of the skin and, by extension, important parameters relevant in determining cardiovascular health and physiological status. These same capabilities can be useful in wound treatment and monitoring during a healing process, cancer screening, core body temperature assessments and others of clinical relevance. In all cases, the ability to wear the devices continuously, over days or weeks, and to perform readout and power delivery via a conventional smartphone, represent uniquely enabling features. Photonic operation in the red and near infrared could enable use in near-surface implantable diagnostics. Fabrication of e-TLC thermal imaging devices The fabrication (details in Supplementary Fig. 1 ) began with spin coating and curing a thin (20 μm) layer of poly(dimethylsiloxane) (PDMS, Sylgard 184, 40:1 mixing ratio) mixed with Iron Oxide Pigment Black 11 (The Earth Pigments Company, LLC) on a substrate of poly(ethyleneterephlatate). A PDMS stamp with arrays of square posts (each post, 0.5 mm × 0.5 mm over an area of 15 cm 2 ; see Supplementary Note 1a ) was contacted against a layer of microencapsulated TLC ink (Hallcrest SSN33R5W). Removing the stamp and drying it in air resulted in the formation of a solid layer of TLC material with an average thickness of 25 μm on the raised regions. A thermal release tape (Nitto Denko REVALPHA 90 °C) facilitated transfer of this material from the stamp to the surface of the black PDMS film. The device was completed by spin coating and curing a thin (30 μm) layer of transparent PDMS on top of the structure, as an encapsulant. Fabrication of the wireless heater for the active e-TLC devices began with spin coating of a thin film of polyimide (Sigma Aldrich) on a sacrificial layer of poly(methylmethacrylate) (100 nm, MicroChem) on a silicon wafer. Metal-evaporation (Cr/Au, 5 nm/50 nm), photolithography and wet-etching defined the serpentine structure for the Joule heater. Additional polyimide spin coating, oxygen reactive-ion etching and metal deposition for contacts, interconnects and antenna circuits completed the wireless system. Dissolving the poly(methylmethacrylate) and then physically transferring the electronic structure to the back side of the e-TLC device completed the fabrication. Device calibration and test for noise level An e-TLC device was placed on a metal plate with black matt finish on a hotplate. Two white fluorescent light sources were placed on opposite sides of the device for illumination in a manner that avoided specular reflection. A digital camera (Canon Mark II 5D) and an infrared camera (FLIR ExaminIR) placed side-by-side were focused on the same area of the device at a distance of ~30 cm. The angle between the cameras and each of the light sources was ~90°. The device was heated to 40 °C on the hotplate and then the hotplate was turned off. During the cooling process, high-resolution images were collected every 10 s with the digital camera; the infrared camera captured frames at a rate of 12.5 s −1 . The process of cooling from 40 °C to 32 °C lasted about 20 min. The colour information of the TLC was extracted from 33 °C to 39°C with steps of 0.5 °C. The set of algorithms developed to accomplish this task are based on computer vision OpenCV ( http://opencv.org/ ) library. The main functions are (in alphabetic order) as follows: ‘adaptiveThreshold’, ‘cvtColor’, ‘dilate’, ‘drawContours’, ‘erode’, ‘findContours’, ‘GaussianBlur’, ‘getStructuringElement’, ‘imread’, ‘inRange’, ‘matchShapes’, ‘minEnclosingCircle’ and ‘threshold’. In HSV colour space, the light intensity information is stored in the ‘value’ channel and is completely separated from the colour information, which is encoded in the ‘hue’ and the ‘saturation’ channels. Hue and saturation are, therefore, a natural basis for temperature calibration, as they are not strongly affected by the change in illumination intensity. Temperature calibration was constructed by means of two-dimensional linear fit. The core function used in the process was ‘lstsq’ from the linear algebra module of Numerical Python ( http://www.numpy.org/ ). Any combination of hue/saturation values can be assigned to a temperature value. Even for materials that are not temperature sensitive, such as the calibration colour pixels, their hue/saturation can be treated as a specific temperature for consistency of analysis. To test the noise level and precision of the system, the hotplate temperature was set at a fixed value; temporal fluctuations of TLC colour, calibration dot colour and infrared emission were recorded using the two cameras over a period of 15 min. The colour changes were converted to temperature fluctuation and compared with infrared fluctuation directly. Reactive hyperaemia test A volunteer (female, 27 years old) reclined in a chair with her left forearm secured gently to an arm rest using Velcro strips to reduce movement. A pressure cuff was secured around the subject’s left bicep. An e-TLC device was placed on the skin of the left wrist approximately above the ulnar artery. Applying puffs of compressed air ensured full, conformal contact. Infrared and digital cameras placed 30 cm above the subject’s left wrist were focused on the location of the device while illuminated with white fluorescent lights. The subject was instructed to relax for 5 min. The cuff was inflated to a pressure of 250 mm Hg for 160 s. Continuous high-resolution colour images and infrared temperature measurements were then collected with the two cameras as the occlusion started and was then released. The total duration of the measurement was 300 s. Experiments were conducted with informed consent of human subjects and in accordance with the ethical guidelines of the National Institutes of Health and with the approval of the Institutional Review Board Office of University of Illinois at Urbana–Champaign. Thermal conductivity/diffusivity and hydration measurements Thermal conductivity was determined by analysing the spatial distribution of temperature for a few seconds immediately after activation of a Joule heater in an active e-TLC device. To validate the computational models, an active e-TLC device was floated on the surface of a mixture of ethylene glycol/water preheated to ~33 °C. A constant voltage supplied to the e-TLC Joule heating element created a steady-state temperature rise of a few degrees at the location of the heater. Images were then collected with a digital and infrared camera set up above the device with only white fluorescent light sources. The spatial decay of temperature in the e-TLC was recorded by analysis of images from the infrared camera and from colour images of the device. The same experiment was performed on a volunteer’s forearm skin. Here, different hydration levels were achieved by applying various amounts of lotion to the measurement location, before application of the active e-TLC device. Immediately after image capture, the e-TLC device was removed and a hydration meter was used to determine the actual moisture level (averaged from five readings). Measurements of thermal diffusivity used a wireless, active e-TLC, with a transmission antenna located ~10 cm away and adjusted to achieve a peak change in temperature of a few degrees (RF power below 2.5 W kg −1 at frequencies between 1.95 and 2.35 GHz, tuned to match the response of the receiver antenna on the e-TLC). Both digital and infrared cameras were focused on the device with a distance of 30 cm. Videos with 60-s duration recorded the changes in temperature associated with activation and de-activation of the heater. The experiment was validated using the ethylene glycol/water system and then repeated on skin with different hydration levels, in procedures otherwise similar to those for the thermal conductivity measurements. How to cite this article: Gao, L. et al . Epidermal photonic devices for quantitative imaging of temperature and thermal transport characteristics of the skin. Nat. Commun. 5:4938 doi: 10.1038/ncomms5938 (2014).